Conserved sequence-specific lincRNA–steroid receptor interactions drive transcriptional repression and direct cell fate The majority of the eukaryotic genome is transcribed, generating a significant number of long intergenic noncoding RNAs (lincRNAs). Although lincRNAs represent the most poorly understood product of transcription, recent work has shown lincRNAs fulfill important cellular functions. In addition to low sequence conservation, poor understanding of structural mechanisms driving lincRNA biology hinders systematic prediction of their function. Here we report the molecular requirements for the recognition of steroid receptors (SRs) by the lincRNA growth arrest-specific 5 (Gas5), which regulates steroid-mediated transcriptional regulation, growth arrest and apoptosis. We identify the functional Gas5-SR interface and generate point mutations that ablate the SR–Gas5 lincRNA interaction, altering Gas5-driven apoptosis in cancer cell lines. Further, we find that the Gas5 SR-recognition sequence is conserved among haplorhines, with its evolutionary origin as a splice acceptor site. This study demonstrates that lincRNAs can recognize protein targets in a conserved, sequence-specific manner in order to affect critical cell functions. An emerging phenomenon in biology is the widening gap between the availability of genomic sequences and the functional understanding of the products encoded within [1] . The vast majority of functional research has focused on protein-coding genes, which constitute only 2% of the human genome [2] . Recently, attention has turned to the non-protein-coding elements of the genome and transcriptome. Although some noncoding RNA molecules (ncRNAs) such as small nucleolar and transfer RNAs have well-defined function, the majority of non-ribosomal, nuclear-encoded RNA molecules present in a cell are of unknown function and/or structure [3] . Of these, long intergenic ncRNAs (lincRNAs), defined as intergenic ncRNAs greater than 200 nucleotides in length, remain the most poorly understood product of transcription [4] . lincRNAs have been shown to function in diverse processes such as pluripotency, development, cell cycle, immunity, transcription and apoptosis [5] , [6] , [7] , [8] , [9] . Until recently, conservation of these lincRNAs was considered non-existent; however, emerging studies show higher conservation in lincRNAs than originally perceived, although well below the level of protein-coding exons [5] , [10] , [11] . Consistent with this observation, a recent study searched for similarity between mouse and zebrafish lincRNAs and found only 9.0% of annotated mouse lincRNAs contained detectable sequence homology to whole-genome zebrafish alignments, with most of this conservation clustered in small domains separated by longer stretches of divergent sequence [12] . Remarkably, mammalian lincRNA orthologues were still able to rescue developmental defects in zebrafish caused by specific lincRNA knockouts, indicating lincRNA function can be conserved despite divergent primary sequence [12] . However, the mechanisms by which lincRNA functions are conserved in a rapidly changing sequence space are unclear. The study of such mechanisms requires the identification of functional domains within lincRNAs. Unfortunately, there are currently few lincRNAs with well-characterized function, and still fewer in which functional domains have been identified and characterized. Known lincRNA functional domains include the 5′ terminal region of lincRNA-p21, which interacts with hnRNP K to mediate the p53 response [7] . HOTAIR, a regulator of gene expression and chromatin state, uses a 5′ domain to bind polycomb repressive complex 2, and a 3′ domain to bind the LSD1/CoREST/REST complex [13] . Another lincRNA, growth arrest-specific 5 (Gas5), uses a region in its 12th exon to interact with and repress the steroid hormone receptors (SRs) [14] . Without detailed structural information about these protein–lincRNA interactions, the basis of conservation (or lack thereof) within lincRNA functional domains is impossible to determine. By focusing on the interaction between SRs and Gas5, we sought to determine the molecular and structural requirements of a particularly important lincRNA–protein interaction. The GAS5 gene is a noncoding 5′ terminal oligo-pyrimidine gene consisting of 12 exons in humans and forms two mature fully-spliced and polyadenylated isoforms in addition to numerous expressed sequence tags [14] , [15] . The 11 introns of the GAS5 gene contain ten box C/D snoRNA genes, which are critical for ribosome modification and embryonic development [16] . Gas5 is present in all tissue types and is one of the most highly expressed noncoding RNAs in the human genome [17] . Gas5 has been implicated in many important cellular and physiological processes, including p53 signalling [7] , embryogenesis [6] , growth arrest and cell cycle [18] , [19] , and apoptosis [14] , [20] , [21] , [22] . In addition, Gas5 is required for rapamycin action in immune cells [20] , and Gas5 knockdown affects mRNA levels for M-Ras, prion protein, parkin and other genes [6] . Gas5 inhibits the transcriptional activity of steroid receptors (SRs) through direct competition for DNA binding [14] . The SR-binding site was previously mapped to a putative stem-loop region (bases 546–566) and described as a ‘mimic’ of genomic SR-binding sites, or glucocorticoid response elements (GREs) [14] . This GRE mimic (GREM) within Gas5 represents a compact lincRNA–protein interaction domain, optimal for examining the effects of altered lincRNA sequence and structure on protein–RNA interactions, and the downstream consequences on cellular processes. Here we describe detailed studies of the mechanistic, structural and evolutionary aspects of the SR–Gas5 interaction. The Gas5 GREM selectively binds 3-keto SRs To measure the binding affinity between glucocorticoid receptor (GR) and Gas5, we monitored via fluorescence polarization (FP) the ability of full-length Gas5 and shorter GREM-containing constructs ( Supplementary Fig. 1 ) to compete with fluorescently labelled DNA-activating GREs, or (+)GREs, for binding to the GR DNA-binding domain (DBD; Fig. 1a ). Full-length Gas5 competed for DNA binding the most strongly, with a K i of 158 nM—within the range of affinities of GR for (+)GREs (80 nM–1 μM) [23] . Shorter constructs ( Supplementary Fig. 1 ) containing only the GREM were sufficient for DNA competition, although affinity was lowered approximately fivefold compared with the full-length Gas5 transcript ( Fig. 1a ). In addition, a fluorescently labelled Gas5 GREM construct containing only the stem bound directly to GR, indicating that only the putative double helical region within the GREM is required for GR binding ( Fig. 1b ), much like GR—DNA binding requires a short, double helical response element. 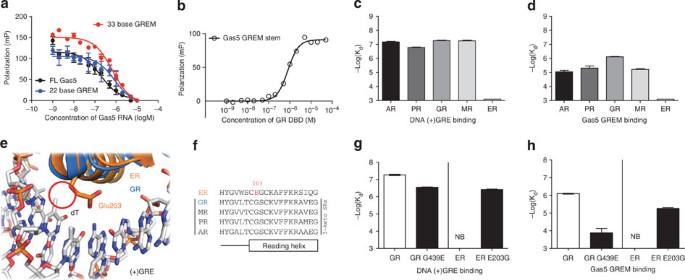Figure 1: Gas5 selectively binds the 3-keto steroid receptors. (a) Full-length Gas5 competes strongly for DNA binding to the glucocorticoid receptor (GR;Ki=158 nM, fit to a one-site binding competition model). Shorter Gas5 constructs (Supplementary Fig. 1) containing only the GREM stemloop are sufficient for GR binding (Kifor the 23 and 33 base constructs are 825 and 654 nM, respectively). Error is shown as ±s.e.m., and was normalized to the mean for figures showing −logKd. (b) A double helical region containing only the GREM stem is sufficient for direct GR binding (Kd=801 nM, fit to a one-site specific binding model). (c) The 3-keto steroid receptors but not the estrogen receptor are able to bind to an activating DNA glucocorticoid response element ((+)GRE). (d) Similarly, the GREM stem construct shown inbbinds the 3-keto steroid receptors, but not the estrogen receptor. However, the estrogen receptor is capable of binding its own response element (Supplementary Fig. 1m). (e) GR and ER recognize their cognate DNA response elements via different sequence-specific contacts. Notably, ER contains a glutamic acid at position 203 (Gly439 in GR), which excludes binding to an activating GR response element, or (+)GRE (f). (g) Mutation of this residue (Glu203) to the homologous GR residue (E203G) restores ER binding to a GRE (right), and the converse mutation in GR (left, G439E) reduces affinity for a GRE. NB, no binding. (h) Remarkably, the ER E203G mutation confers binding to Gas5 (right), demonstrating that Gas5 exploits differences in GR/ER nucleic acid specificity to selectively target the non-ER steroid receptors. Binding experiments were performed in duplicate (full-length Gas5, panela) or triplicate (all others), with three internal replicates each. Figure 1: Gas5 selectively binds the 3-keto steroid receptors. ( a ) Full-length Gas5 competes strongly for DNA binding to the glucocorticoid receptor (GR; K i =158 nM, fit to a one-site binding competition model). Shorter Gas5 constructs ( Supplementary Fig. 1 ) containing only the GREM stemloop are sufficient for GR binding ( K i for the 23 and 33 base constructs are 825 and 654 nM, respectively). Error is shown as ±s.e.m., and was normalized to the mean for figures showing −logK d . ( b ) A double helical region containing only the GREM stem is sufficient for direct GR binding ( K d =801 nM, fit to a one-site specific binding model). ( c ) The 3-keto steroid receptors but not the estrogen receptor are able to bind to an activating DNA glucocorticoid response element ((+)GRE). ( d ) Similarly, the GREM stem construct shown in b binds the 3-keto steroid receptors, but not the estrogen receptor. However, the estrogen receptor is capable of binding its own response element ( Supplementary Fig. 1m ). ( e ) GR and ER recognize their cognate DNA response elements via different sequence-specific contacts. Notably, ER contains a glutamic acid at position 203 (Gly439 in GR), which excludes binding to an activating GR response element, or (+)GRE ( f ). ( g ) Mutation of this residue (Glu203) to the homologous GR residue (E203G) restores ER binding to a GRE (right), and the converse mutation in GR (left, G439E) reduces affinity for a GRE. NB, no binding. ( h ) Remarkably, the ER E203G mutation confers binding to Gas5 (right), demonstrating that Gas5 exploits differences in GR/ER nucleic acid specificity to selectively target the non-ER steroid receptors. Binding experiments were performed in duplicate (full-length Gas5, panel a ) or triplicate (all others), with three internal replicates each. Full size image Previous work demonstrated that Gas5 regulates the transcriptional activity of not only GR, but also the androgen receptor (AR), progesterone receptor (PR) and mineralocorticoid receptor (MR), which share the ability to bind 3-keto steroids as well as DNA (+)GREs [14] . Other nuclear receptors such as the estrogen receptor (ER), peroxisome proliferator-activated receptor (PPAR) and retinoid X receptor (RXR), which bind different DNA response elements, are not susceptible to Gas5-mediated repression [14] . To determine the relative affinity of the Gas5 GREM for all SRs, we tested the ability of recombinantly expressed DBDs from all five SRs to bind both (+)GRE DNA and the Gas5 GREM stem ( Fig. 1c,d ). All 3-keto SRs bound both to a DNA (+)GRE and to the Gas5 GREM, which is consistent with their transcriptional repression by Gas5 (ref. 14 ). As predicted, the ER DBD bound only to an ER response element (ERE), and was unable to bind the Gas5 GREM ( Fig. 1c,d , Supplementary Fig. 1m,n ). Gas5 exploits sequence differences among protein targets Given their similar structure and sequence (>50% identity within the DBD), it is unclear how Gas5 discriminates among SRs; for example, the ER and GR DBDs share an identical fold and insert an α-helix to read the major groove of DNA ( Fig. 1e ). However, key amino-acid differences in this helix allow the two receptors to bind disparate response elements. Notably, one ER side chain, Glu203, makes contact with DNA when bound to an ERE, whereas the 3-keto SRs contain a glycine at this position ( Fig. 1f ). When bound to a ERE, ER Glu203 contacts a cytosine, forming an interaction required for DNA binding and subsequent gene activation [24] . The 3-keto SRs do not contact DNA at this position, and substitution of glycine with a bulkier amino-acid side chain would introduce steric clashes with (+)GRE DNA bases ( Fig. 1e ). Remarkably, mutation of this single amino acid in ER to glycine (E203G) confers ER binding not only to a DNA (+)GRE ( Fig. 1g ), but also to the Gas5 GREM ( Fig. 1h ). Likewise, the converse mutation in GR (G439E) reduced GR binding to both a DNA (+)GRE and the Gas5 GREM ( Fig. 1g,h ). The discrimination among evolutionary-related proteins by Gas5 demonstrates that lincRNAs are capable of sequence-specific interactions with their target proteins. In addition, the strong correlation between DNA binding and Gas5 RNA binding suggest the presence of sequence-specific, (+)GRE-like SR contacts in the Gas5 major groove. A widened major groove facilitates GREM-SR binding Previous work postulated that a putative double-helical region of the GREM mediated SR-Gas5 binding [14] . Ultraviolet melting experiments confirm that the Gas5 GREM stemloop indeed forms a secondary structure in solution ( T m =58 °C; Supplementary Fig. 2a ). To determine the local RNA structure required for Gas5-SR recognition, we determined the X-ray crystal structure of the Gas5 GREM stem to a resolution of 1.9 Å. Two merohedrally twinned crystal forms were obtained in the rhombohedral space group R3, but twin refinement yielded excellent electron density and statistics ( Table 1 , Supplementary Table 1 , and Supplementary Fig. 2b ). In both crystal forms, the Gas5 GREM adopts an A-form double helix with a widened major groove. The average minor and major grooves widths are greater than 15.0 Å in both crystal structures; wider than most A-form RNA helices found in crystal structures, but within the broader range of major groove widths in solution as determined by NMR [25] . GR-bound DNA response elements of GR exhibit major groove widths approximately 1.5–3.0 Å wider than the free Gas5 GREM structure [23] , [26] , indicating that only minimal secondary structure perturbation may be necessary for GR-Gas5 binding ( Supplementary Fig. 2c,d ). Table 1 Data collection and refinement statistics for Gas5 GREM X-ray crystal structures. Full size table Molecular determinants and model of the GR–Gas5 interaction To identify bases within the GREM for critical SR–Gas5 binding, we performed hydroxyl radical footprinting and used NMR to structurally map the GR–Gas5 interaction. Increasing concentrations of GR DBD protected several portions of the GREM stem from OH· hydrolysis while deprotecting bases U554-U556 within the loop ( Fig. 2a–c ). The pattern of protection indicates GR interaction with the major groove, much like its classical interaction with DNA. To visualize the impact of GR binding on Gas5, we obtained two-dimensional homonuclear [ 1 H, 1 H] nuclear Överhauser enhancement spectroscopy (NOESY) spectra via 1 H NMR of the Gas5 GREM stemloop both in the presence and absence of the GR DBD ( Fig. 2d–f ). Nucleotides within the Gas5 GREM stem showed NMR resonances with moderate or strong line broadening upon addition of GR DBD, whereas others displayed strongly shifted positions (>0.025 p.p.m.). Broadened resonances correspond to nucleotides that are switching between two states in the intermediate exchange NMR timescale, whereas resonances that are simultaneously shifted and broadened are switching between two states in the slow-to-intermediate or intermediate-to-fast exchange regime. Only C561 and U569 have H1′-H6 resonances that are shifted but not broadened, and therefore, have two states that are in slow or fast exchange. The two states may correspond to nucleotides situated in disparate chemical shift environments, such as (i) free versus GR DBD-bound Gas5 RNA, (ii) two Gas5 RNA conformational states in the presence of GR DBD or (iii) as a result of interactions with a neighbouring Gas5 RNA or with another Gas5 RNA region within the same molecule. Both NMR and OH· footprinting demonstrated conformational changes in the four base loop upon GR binding ( Fig. 2c ), consistent with previous studies indicating that bulges and loops can widen the RNA major groove, presenting surfaces for protein interaction [27] , [28] . 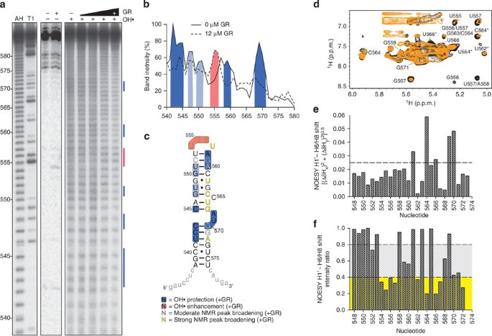Figure 2: Base-specific interactions mediate the glucocorticoid receptor–Gas5 interaction. (a) GR protects the Gas5 GREM from OH· hydrolysis. Increasing amounts of GR DBD were added toin vitrotranscribed Gas5 GREM RNA and subjected to OH· hydrolysis, followed by denaturing polyacrylamide gel electrophoresis; a representative gel is shown. GR-mediated protection from OH· hydrolysis is quantified inb. Light and dark blue indicate moderate and strong protection (>±10% and 20%, respectively) with GR DBD, and red indicates deprotection in the presence of GR DBD. (c) Results from NMR and OH· footprinting are mapped onto the Gas5 GREM. (d) Zoomed in overlay of free Gas5 RNA (black) and 1:1 Gas5 RNA:GR DNA-binding domain (DBD; orange) 2D [1H,1H]-NOESY spectra with 200 ms mixing time. Broadened resonances in the presence of GR DBD are labelled. Intra-nucleotide H1’-H6/H8 resonances are labelled according to nucleotide type and position number. H5-H6 peaks are labelled in the same way, followed by an asterisk (*). Peak labels separated by a slash (/) are for inter-nucleotide H1’-H6/H8 NOESY crosspeaks. (e) NMR crosspeak shifting calculated from NOESY spectra for free and GR DBD-bound Gas5 GREM stem reveals strongly shifted resonances (changes >0.025 p.p.m.; horizontal dashed line). (f) NMR crosspeak line broadening determined from NOESY spectra as calculated from the crosspeak intensity ratio for free and GR-DBD-bound Gas5 GREM stem (‘moderately broadened’ resonances, >0.4, grey; ‘strongly broadened’ resonances, >0.8, yellow). Figure 2: Base-specific interactions mediate the glucocorticoid receptor–Gas5 interaction. ( a ) GR protects the Gas5 GREM from OH· hydrolysis. Increasing amounts of GR DBD were added to in vitro transcribed Gas5 GREM RNA and subjected to OH· hydrolysis, followed by denaturing polyacrylamide gel electrophoresis; a representative gel is shown. GR-mediated protection from OH· hydrolysis is quantified in b . Light and dark blue indicate moderate and strong protection (>±10% and 20%, respectively) with GR DBD, and red indicates deprotection in the presence of GR DBD. ( c ) Results from NMR and OH· footprinting are mapped onto the Gas5 GREM. ( d ) Zoomed in overlay of free Gas5 RNA (black) and 1:1 Gas5 RNA:GR DNA-binding domain (DBD; orange) 2D [ 1 H, 1 H]-NOESY spectra with 200 ms mixing time. Broadened resonances in the presence of GR DBD are labelled. Intra-nucleotide H1’-H6/H8 resonances are labelled according to nucleotide type and position number. H5-H6 peaks are labelled in the same way, followed by an asterisk (*). Peak labels separated by a slash (/) are for inter-nucleotide H1’-H6/H8 NOESY crosspeaks. ( e ) NMR crosspeak shifting calculated from NOESY spectra for free and GR DBD-bound Gas5 GREM stem reveals strongly shifted resonances (changes >0.025 p.p.m. ; horizontal dashed line). ( f ) NMR crosspeak line broadening determined from NOESY spectra as calculated from the crosspeak intensity ratio for free and GR-DBD-bound Gas5 GREM stem (‘moderately broadened’ resonances, >0.4, grey; ‘strongly broadened’ resonances, >0.8, yellow). Full size image To map the surface through which GR interacts with Gas5, we collected two-dimensional [ 1 H, 15 N]-heteronuclear single quantum coherence (HSQC) data on the GR DBD both free and bound to the Gas5 GREM ( Fig. 3a–c ). Notably, chemical shift perturbations are observed in helix 1 of the DBD when bound to either DNA [29] or Gas5 RNA, indicating that GR uses its DNA-binding interface to bind RNA ( Fig. 3b–e ). Additional regions of the GR DBD that contact DNA in a nonspecific manner, such as helix 2 and the N-terminus, are also perturbed when GR is bound to DNA and RNA. However, no chemical shift perturbations are observed in the dimerization interface (‘D-loop’) of the DBD upon RNA binding as is observed with GR DBD–(+) GRE interactions [30] , providing no evidence for dimerization on RNA ( Fig. 3c,e ). These GR DBD [ 1 H, 15 N]-HSQC data, Gas5 GREM [ 1 H, 1 H] NOESY spectra and mutagenesis data were used to generate a model of the GR DBD–Gas5 GREM complex using HADDOCK [31] . In line with the hypothesis that the Gas5 GREM is a RNA mimic of DNA response elements, the top scoring models showed the GR DBD reading the Gas5 GREM by inserting helix 1 into the major groove ( Fig. 4a ). 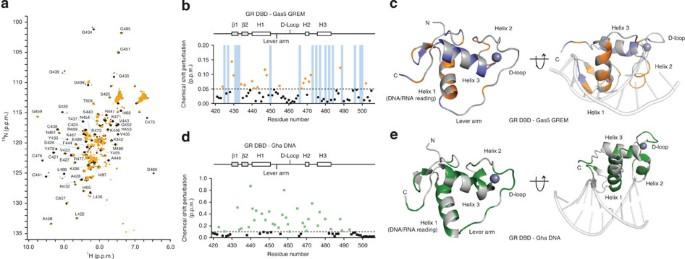Figure 3: NMR reveals that Gas5 interacts directly with residues that comprise GR’s DNA-binding interface. (a) 2D [1H,15N]-HSQC spectra of GR DBD free (black) and bound to the Gas5 GREM (orange). (b) Chemical shift perturbations induced in GR DBD upon binding Gas5. Perturbations greater than 0.05 p.p.m. are coloured orange; blue vertical lines represent resonances that broaden upon binding Gas5 and are no longer observed. (c) GR chemical shift perturbations upon GREM binding mapped onto the HADDOCK model of GR DBD bound to the Gas5 GREM. (d) Chemical shift perturbations greater than 0.1 p.p.m. (green) induced in GR DBD upon binding Gha DNA29plotted against GR DBD primary and secondary structure. (e) GR chemical shifts upon Gha DNA binding mapped onto the GR DBD crystal structure (PDB 4HN5). Figure 3: NMR reveals that Gas5 interacts directly with residues that comprise GR’s DNA-binding interface. ( a ) 2D [ 1 H, 15 N]-HSQC spectra of GR DBD free (black) and bound to the Gas5 GREM (orange). ( b ) Chemical shift perturbations induced in GR DBD upon binding Gas5. Perturbations greater than 0.05 p.p.m. are coloured orange; blue vertical lines represent resonances that broaden upon binding Gas5 and are no longer observed. ( c ) GR chemical shift perturbations upon GREM binding mapped onto the HADDOCK model of GR DBD bound to the Gas5 GREM. ( d ) Chemical shift perturbations greater than 0.1 p.p.m. (green) induced in GR DBD upon binding Gha DNA [29] plotted against GR DBD primary and secondary structure. ( e ) GR chemical shifts upon Gha DNA binding mapped onto the GR DBD crystal structure (PDB 4HN5). 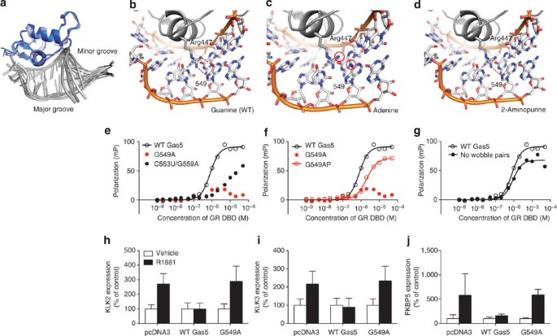Figure 4: A single-nucleotide mutation within Gas5 eliminates its ability to bind steroid receptors and repress steroid-driven transcription. (a) Superposition of the highest-scoring cluster of GR–Gas5 GREM models generated by HADDOCK. In these models, GR binds in the major groove to the A-form helix of the Gas5 GREM. (b) Guanine 549 presents a carbonyl moiety towards the major groove, which GR may recognize with a basic amino acid such as Arg447 (modelled here by HADDOCK) or Lys442. (c) Mutation of guanine 549 to adenine introduces an amine in the major groove, which would clash with the basic major-groove reading amino acids of GR. However, mutation of this guanine to 2-aminopurine (d) removes this carbonyl moiety without affecting the minor groove interaction surface. (e) Mutation of the two guanine bases, including position 549, identified by structure probing (Fig. 2) to adenine ablates binding of GR to the Gas5 GREM stem. Binding (e–g) data are fit to a one-site specific binding model. (f) The G549A mutation ablates GR binding to the Gas5 GREM stem. However, mutation of G549 to 2-aminopurine reduces GR–Gas5 GREM stem binding only 2.5-fold, indicating that GR contacts the major groove of Gas5 (seeb–d). (g) Two G-U wobble pairs (including G549) are present in the GREM; however, Watson–Crick G-C pairs are also compatible with GR binding. (h–j) The G549A mutation, which ablates SR-Gas5 bindingin vitro, also compromises Gas5-mediated repression of steroid-driven transcriptional activation in 22Rv1 cells. Three androgen receptor-responsive genes were measured and normalized toACTBvia reverse transcription PCR (RT–PCR) in 22Rv1 prostate cancer cells with and without the AR agonist R1881. In all panels, error is shown as ±s.e.m, and binding experiments and RT–PCR were both performed in triplicate. Full size image Figure 4: A single-nucleotide mutation within Gas5 eliminates its ability to bind steroid receptors and repress steroid-driven transcription. ( a ) Superposition of the highest-scoring cluster of GR–Gas5 GREM models generated by HADDOCK. In these models, GR binds in the major groove to the A-form helix of the Gas5 GREM. ( b ) Guanine 549 presents a carbonyl moiety towards the major groove, which GR may recognize with a basic amino acid such as Arg447 (modelled here by HADDOCK) or Lys442. ( c ) Mutation of guanine 549 to adenine introduces an amine in the major groove, which would clash with the basic major-groove reading amino acids of GR. However, mutation of this guanine to 2-aminopurine ( d ) removes this carbonyl moiety without affecting the minor groove interaction surface. ( e ) Mutation of the two guanine bases, including position 549, identified by structure probing ( Fig. 2 ) to adenine ablates binding of GR to the Gas5 GREM stem. Binding ( e – g ) data are fit to a one-site specific binding model. ( f ) The G549A mutation ablates GR binding to the Gas5 GREM stem. However, mutation of G549 to 2-aminopurine reduces GR–Gas5 GREM stem binding only 2.5-fold, indicating that GR contacts the major groove of Gas5 (see b – d ). ( g ) Two G-U wobble pairs (including G549) are present in the GREM; however, Watson–Crick G-C pairs are also compatible with GR binding. ( h – j ) The G549A mutation, which ablates SR-Gas5 binding in vitro , also compromises Gas5-mediated repression of steroid-driven transcriptional activation in 22Rv1 cells. Three androgen receptor-responsive genes were measured and normalized to ACTB via reverse transcription PCR (RT–PCR) in 22Rv1 prostate cancer cells with and without the AR agonist R1881. In all panels, error is shown as ±s.e.m, and binding experiments and RT–PCR were both performed in triplicate. Full size image A single GREM mutation abolishes the SR–Gas5 interaction The specificity of GR and 3 keto-SR-DNA recognition is heavily dictated by the contact of arginine and lysine residues in helix 1 of the GR DBD with two guanine-cytosine (GC) pairs in the (+)GRE major groove. Surprisingly, two equivalently spaced guanine-containing pairs (G549 and G559) are present in the Gas5 RNA GREM and were identified by structure probing as participating in the GR–Gas5 interaction ( Fig. 2 ). Mutating these two guanines to adenine, which replaces the major groove O6 carbonyl with an amine, ablates GR binding ( Fig. 4b–f ). Mutation of G549 to 2-aminopurine, which selectively removes a potential hydrogen bond acceptor (O6) from the major groove while leaving the minor groove unchanged, diminishes but does not abolish binding. Critically, these Gas5 RNA mutations preserve secondary structure as monitored by ultraviolet melting ( Supplementary Table 2 ). Along with the structural data above, these experiments establish that GR indeed binds Gas5 in the major groove. In addition, protein recognition of RNA wobble pairs has been reported in several systems [32] , [33] , and two such non-Watson–Crick interactions are present in the Gas5 GREM: U548-G563 and G549-U562. To determine whether GR-GREM recognition depends on this wobble base pairing, we mutated these G-U pairs to canonical Watson–Crick G-C pairs. This mutation only marginally affected GR binding ( Fig. 4g ), indicating that GR does not discriminate between guanine-uracil and guanine-cytosine pairs. To examine the effect of the G549A mutation on SR-mediated transcription in cells, we transfected AR-positive 22Rv1 prostate cancer cells, with wild-type (WT) Gas5, Gas5 with the G549A mutation or empty vector (pcDNA3.1). In these cells, WT Gas5 inhibited the androgen-driven expression of several AR target genes ( Fig. 4h–j ). However, this effect was reversed by the G549A mutation, with expression of the AR target genes returning to vector control levels. We therefore identified a single-nucleotide mutation is sufficient to ablate the interaction between SRs and Gas5 both in vitro and in cells. The Gas5 G549A mutant prevents Gas5-induced apoptosis Gas5 is downregulated in both breast and prostate cancers, and its reintroduction accelerates apoptosis in both prostate and breast cancer cell lines [21] , [22] , [34] . However, the potential role of the Gas5–SR interaction in cancer cell proliferation and survival has not been studied. To test whether a Gas5 mutant specifically compromised in SR interaction displays aberrant function in SR-driven cancer cell lines, we tested the ability of both the WT and G549A Gas5 to drive apoptosis when expressed in 22Rv1 prostate cancer cells. Transfection of both the WT and mutant constructs increased Gas5 expression compared with the vector control ( Fig. 5a ), but only the WT sequence caused caspase activation in these cells, and this was accompanied by a corresponding decrease in cell viability ( Fig. 5b,c ). The G549A mutant, in contrast, had no effect on either parameter ( Fig. 5b,c ). We repeated these experiments in the PR + /ER + breast cancer cell line MCF-7; again, the G549A mutant completely prevented the pro-apoptotic phenotype induced by transfection of WT Gas5 ( Fig. 5d–f ). Thus, in steroid-driven cancer cells such as 22Rv1 cells, Gas5 function appears to be directly related to the SR-Gas5 signalling axis. 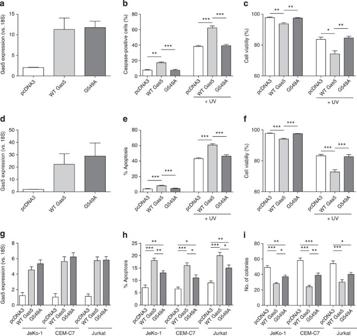Figure 5: Selective ablation of the steroid receptor–Gas5 interaction has dramatic effects on cell fate. (a) Quantification of Gas5 levels normalized to 18S RNA in 22Rv1 cells after transfection with WT Gas5, G549A Gas5 and pcDNA3 constructs. (b) WT Gas5 induces caspase-dependent cell death in 22Rv1 cells, but this effect is completely reversed in the G549A mutant. Similar effects were seen for cell viability (c). (d)MCF-7 cells were transfected with identical constructs, and levels quantified via reverse transcription PCR and normalized to 18S RNA. The G549A mutation completely ablated the pro-apoptotic (e) effects and reduction in cell viability (f) caused by transfection of WT Gas5. (g) Likewise, three suspension cell lines were transfected with pcDNA3, WT Gas5 or the G549A mutant and expression were quantified as above. In these cell lines, the G549A mutation only partially reverses the apoptotic effects (h) and colony-forming effects (i) seen by transfection of WT Gas5. For all panels, experiments were performed in triplicate, and error is shown as ±s.e.m. and was normalized to the mean for figures showing –logKd. One, two and three asterisks indicateP<0.05, 0.01 and 0.001, respectively by one-way ANOVA with Tukey’spost-hoctest. Figure 5: Selective ablation of the steroid receptor–Gas5 interaction has dramatic effects on cell fate. ( a ) Quantification of Gas5 levels normalized to 18S RNA in 22Rv1 cells after transfection with WT Gas5, G549A Gas5 and pcDNA3 constructs. ( b ) WT Gas5 induces caspase-dependent cell death in 22Rv1 cells, but this effect is completely reversed in the G549A mutant. Similar effects were seen for cell viability ( c ). ( d) MCF-7 cells were transfected with identical constructs, and levels quantified via reverse transcription PCR and normalized to 18S RNA. The G549A mutation completely ablated the pro-apoptotic ( e ) effects and reduction in cell viability ( f ) caused by transfection of WT Gas5. ( g ) Likewise, three suspension cell lines were transfected with pcDNA3, WT Gas5 or the G549A mutant and expression were quantified as above. In these cell lines, the G549A mutation only partially reverses the apoptotic effects ( h ) and colony-forming effects ( i ) seen by transfection of WT Gas5. For all panels, experiments were performed in triplicate, and error is shown as ±s.e.m. and was normalized to the mean for figures showing –logK d . One, two and three asterisks indicate P <0.05, 0.01 and 0.001, respectively by one-way ANOVA with Tukey’s post-hoc test. Full size image The expression of Gas5 variants has differential effects in immune cells, which are less dependent on SR signalling for growth [18] . To determine the role of SR-Gas5 interactions in apoptosis and viability in these cells, we transfected three suspension cell lines, JeKo-1, CEM-C7 and Jurkat, with the WT and G549A Gas5 constructs ( Fig. 5g ). Among all three cell lines, transfection of WT Gas5 induced apoptosis and a corresponding decrease in cell viability ( Fig. 5h,i ) as we previously reported [18] . Interestingly, the G549A mutation only partially reversed this phenotype (Fig. 5h,i), in contrast to the complete reversal of apoptosis induction seen in steroid-driven cancer cell lines ( Fig. 5b–c,e–f ). These results indicate that Gas5 has functions beyond regulating SRs, such as mediating mammalian target of rapamycin signalling [20] , and additional regions of the Gas5 transcript play important roles in regulating apoptosis in immune cells. GR cannot bind its own transcribed genomic binding sites As 70% of the genome is transcribed, there may be many Gas5-like RNAs capable of binding and modulating the activity of SRs. In particular, there are ~2.3 × 10 6 genomic sequences matching a GR-binding motif [35] , and many of these lie within transcribed regions. Owing to their inverted repeat sequence, transcribed (+)GREs could form a stemloop structure much like the Gas5 GREM ( Fig. 6a ), which led us to inquire whether a RNA GREM could readily evolve from a DNA GR-binding site. However, a (+)GRE-derived stemloop differs from the Gas5 GREM in two ways. First, the loop of the (+)GRE structure would contain a 3-base loop, whereas the GREM contains a 4-base loop. Second, the (+)GRE sequence differs slightly from the bases found in the Gas5 GREM ( Fig. 6a ). 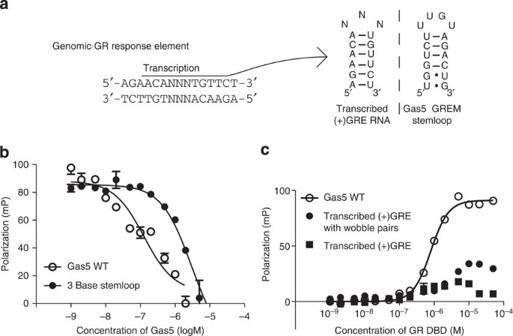Figure 6: The glucocorticoid receptor will not bind its transcribed genomic response elements. (a) Within genomic DNA, GR binds (+)GREs, which are inverted repeats separated by three nucleotides. Such inverted repeat sequences would form a stemloop with similar sequence to the Gas5 GREM when transcribed (on right). However, this sequence is incapable of binding GR because of both secondary structure constraints caused by a three-base stemloop (b) as well as a different primary sequence (c). (b) Competition for a fluorescently labelled (+)GRE DNA construct was performed with a WT GREM-containing 51nt construct or an otherwise-identical construct with a three-base stemloop (ΔG556). The affinity of the WT construct for GR (Ki) was 125 nM, similar to that of full-length Gas5 (Fig. 1a). (c) A fluorescently labelled transcribed (+)GRE sequence with Gas5 GREM stem flanking sequences was tested for binding to the GR DBD. Binding (b,c) data are fit to a one-site competition or specific binding model, with error shown as ±s.e.m. Binding experiments were performed in duplicate (b) or triplicate (c), with three internal replicates each. Figure 6: The glucocorticoid receptor will not bind its transcribed genomic response elements. ( a ) Within genomic DNA, GR binds (+)GREs, which are inverted repeats separated by three nucleotides. Such inverted repeat sequences would form a stemloop with similar sequence to the Gas5 GREM when transcribed (on right). However, this sequence is incapable of binding GR because of both secondary structure constraints caused by a three-base stemloop ( b ) as well as a different primary sequence ( c ). ( b ) Competition for a fluorescently labelled (+)GRE DNA construct was performed with a WT GREM-containing 51nt construct or an otherwise-identical construct with a three-base stemloop (ΔG556). The affinity of the WT construct for GR ( K i ) was 125 nM, similar to that of full-length Gas5 ( Fig. 1a) . ( c ) A fluorescently labelled transcribed (+)GRE sequence with Gas5 GREM stem flanking sequences was tested for binding to the GR DBD. Binding ( b , c ) data are fit to a one-site competition or specific binding model, with error shown as ±s.e.m. Binding experiments were performed in duplicate ( b ) or triplicate ( c ), with three internal replicates each. Full size image To test the effects of the decreased-length loop on GR binding, which would occur upon transcription of a (+)GRE, we generated the WT Gas5 GREM with a 3-base loop UUU loop rather than the 4-base UUGU loop found in WT Gas5. Although 3-base loops are often less stable than 4-base loops, a UUU loop with a closing AU pair demonstrates adequate stability [36] . Nonetheless, the 3-base loop Gas5 GREM showed lower affinity for GR than the WT 4-loop structure, indicating that inverted repeat sequences with 3-base spacers are unlikely to be active GR-binding elements following transcription ( Fig. 6b ). However, it is possible that a SR-binding RNA sequence such as the GREM could form via a single-nucleotide insertion into a (+)GRE, creating a 4-base stemloop for SR binding. To eliminate effects of the loop length, we placed the consensus (+)GRE halfsite within the Gas5 GREM stem, which is sufficient for GR binding ( Fig. 1b ). GR could not bind this consensus sequence with either Watson–Crick or Gas5-like wobble pairs ( Fig. 6c ), but required additional two additional nucleotide changes to achieve GR-binding ability ( Supplementary Fig. 3 ). These results indicate that Gas5 independently and convergently evolved a SR-binding surface, perhaps aided by the rapid sequence evolution of lincRNAs compared with coding genes. Such a mechanism, whereby a lincRNA acquires the ability to recognize protein targets could be common, and we sought to establish the evolutionary origin of the Gas5 GREM. The Gas5 GREM evolved from a splice acceptor site The GAS5 gene is annotated in only three genomes in the Ensembl database, and the low sequence conservation of lincRNAs makes sequence alignment across multiple species challenging. Fortunately, human Gas5 hosts ten small nucleolar RNAs (snoRNAs) that are highly conserved throughout vertebrates. Intron 11, just upstream of the Gas5 GREM, contains the snoRNA gene U81 , which is positionally conserved from reptiles to mammals. The length of intronic sequence from snoRNAs to the downstream 3′ acceptor splice site is restricted for proper processing of box C/D snoRNAs, with lengths of 65–75 nucleotides from a box C/D snoRNA to the downstream exon ideal for efficient snoRNA excision [37] . As Gas5-containing snoRNAs are critical for embryonic development [16] , we expected the length of intronic sequence downstream of these snoRNAs to be well conserved. Using this anticipated high conservation of snoRNA sequence and intronic length as a guide, we were able to align the Gas5 GREM sequences from over 40 vertebrates. Gas5 does not appear to be present in jawless fish. As expected, the distance from U81 to the downstream splice acceptor site was tightly clustered across vertebrates ( Fig. 7a ). 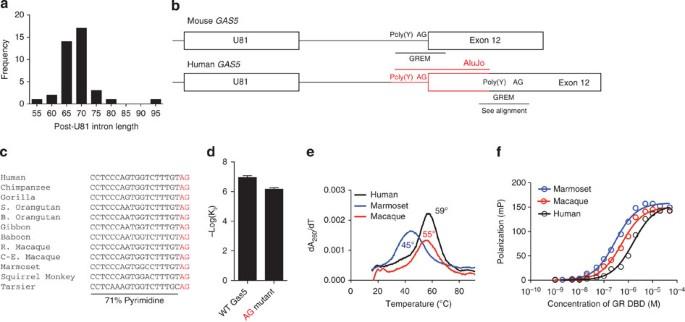Figure 7: The Gas5 GREM evolved from a splice acceptor site. (a) The downstream intron length from the snoRNA U81 is highly conserved because of excision constraints, illustrating the importance of sequence and positional conservation of the splice acceptor site at this locus. (b) The Gas5 GREM was interrupted by an AluJo insertion (red) in haplorhines, moving the ancestral splice acceptor site into exon 12, where splicing no longer occurs. Poly(Y) indicates the position of a polypyrimidine tract. (c) However, despite the lack of splicing at the haplorhine GREM, the haplorhine GREM maintains a splice site-like sequence with a polypyrimidine tract followed by an AG dinucleotide, which is required for high-affinity steroid receptor-Gas5 binding (mutated to GA ind). Other haplorhine species contain Gas5 GREM sequences that exhibit similar secondary structure (e) and GR-binding affinity to the human Gas5 GREM (f). Error is shown as ±s.e.m., and was normalized to the mean for figures showing –logKd. Binding data (f) were fit to a one site, specific binding model. Binding experiments were performed in duplicate (d) or triplicate (f), with three internal replicates each. Figure 7: The Gas5 GREM evolved from a splice acceptor site. ( a ) The downstream intron length from the snoRNA U81 is highly conserved because of excision constraints, illustrating the importance of sequence and positional conservation of the splice acceptor site at this locus. ( b ) The Gas5 GREM was interrupted by an AluJo insertion (red) in haplorhines, moving the ancestral splice acceptor site into exon 12, where splicing no longer occurs. Poly(Y) indicates the position of a polypyrimidine tract. ( c ) However, despite the lack of splicing at the haplorhine GREM, the haplorhine GREM maintains a splice site-like sequence with a polypyrimidine tract followed by an AG dinucleotide, which is required for high-affinity steroid receptor-Gas5 binding (mutated to GA in d ). Other haplorhine species contain Gas5 GREM sequences that exhibit similar secondary structure ( e ) and GR-binding affinity to the human Gas5 GREM ( f ). Error is shown as ±s.e.m., and was normalized to the mean for figures showing –logK d . Binding data ( f ) were fit to a one site, specific binding model. Binding experiments were performed in duplicate ( d ) or triplicate ( f ), with three internal replicates each. Full size image The most striking feature of the GAS5 GREM alignment is the presence of an Alu insertion in the haplorhine lineage, belonging to the AluJo family ( Fig. 7b ). This insertion occurred directly at the GAS5 intron 11/exon 12 boundary, lengthening the GAS5 exon 12 by 100 nucleotides compared with mice. In haplorhines, an Alu-contained splice acceptor site is used for Gas5 transcript processing, maintaining the strict requirement for intron length downstream of U81 . However, this insertion demonstrates that the GREM, although exonic in humans and other haplorhines, evolved from an ancestral splice acceptor site still present in other vertebrates. Multiple previously unassigned cDNAs from GenBank support both the alignment as well as the presence of a splice site at the GREM ( Supplementary Table 3 ). The AluJo insertion re-positioned the ancestral splice acceptor site to be fully contained within exon 12, and it is this now-defunct splice site through which the SRs bind Gas5 ( Fig. 7b ). Owing to snoRNA excision restraints, the haplorhine Gas5 GREM, over 150 bases downstream of U81 , would be under negative selection to lose the ancestral splice site features located inside exon 12 incorporated with the AluJo insertion. However, if this locus was selected for both its splice site sequence and SR-binding ability before the Alu insertion, it is possible that splice-site like sequences required for SR binding would be conserved. Remarkably, when haplorhine GREM sequences are aligned, splice site-like features are readily apparent: a polypyrimidine tract and acceptor AG sequence are conserved throughout the haplorhine clade, despite a lack of splicing at this locus ( Fig. 7c ). The splice site-like sequence shows higher sequence identity among 14 haplorhines (93.8 versus 84.5% for the remainder of exon 12). In addition, relative rate analysis of each position within the ancestral splice site reveals a lower rate of nucleotide substitution within the GREM versus the remainder of exon 12, supporting sequence conservation of the splice site-like sequences required for GR binding to the GREM ( Supplementary Fig. 4 ). Mutation of these splice site-like features, such as the AG within the ancestral splice acceptor sequence, reduces the GREM’s affinity for GR binding ( Fig. 7d ), suggesting that other haplorhines contain conserved, functional GREMs with both a primary sequence and secondary structure capable of binding SRs. Indeed, the GREM sequences of two other haplorhines formed secondary structures in solution ( Fig. 7e ) and were capable of binding the GR DBD ( Fig. 7f ). Given the evolutionary origin of the human Gas5 GREM as a splice acceptor site, it is possible that alternate splicing of the GAS5 gene may control its ability to bind and repress GR in non-haplorhines. The mouse splice isoforms with exon 11 excised or retained bound GR in vitro ( Supplementary Fig. 5a ), and the GREM derived from both the splice or unspliced Gas5 transcripts was sufficient for secondary structure formation and GR binding ( Supplementary Fig. 5b,c ). When we tested for GR–Gas5 binding across the vertebrate clade, eutherian mammals demonstrated the highest affinity interaction ( Supplementary Fig. 5d ), suggesting that the Gas5 GREM was perhaps capable of binding SRs at the time of the AluJo insertion, roughly 55 Mya [38] . However, further study of the mouse and other mammalian Gas5 transcripts is required to definitively determine if GR regulation is a conserved property of Gas5 outside of the haplorhine clade. This is especially true given the short lifetime of unspliced Gas5 and the shorter length of exon 12 in mice compared with haplorhine Gas5 ( Fig. 7b ). Gas5 is retrotransposed within multiple mammalian lineages Finally, given the unique ability of the GREM to bind SRs, we searched for additional GREM-like sequences within the human genome, which could serve as SR-repressing elements. Remarkably, we found processed copies of Gas5 in at least five locations in the human genome, including within the introns of four genes: GABRB3 , NAPEPLD1 , MDN1 and SV2C ( Supplementary Fig. 6 ). At least 29 splice variants of the GAS5 gene are known [15] , and GAS5 retrotransposition events mirror this complexity. Two human copies are fully spliced (splice variant GAS5 -001; Supplementary Fig. 6 ), whereas the sequence within the GABRB3 gene is a copy of the GAS5- 008 splice variant ( Supplementary Fig. 6 ). In addition, some retrotransposed copies of Gas5 are from unreported, species-specific, or ancestral splice variants, such as a copy in gibbons that contains exons 1–4, 6, 7, 11 and 12 ( Supplementary Fig. 6 ). Such a splice variant is not currently described in humans. GAS5 appears to be highly susceptible to retrotransposition, with either full or partial copies of the processed Gas5 present in multiple mammalian lineages, including mice, dogs and more distal members of the mammalian clade, such as sloths ( Supplementary Table 4 ). At least 15 independent copies appear in the haplorhine lineage with many of these copies located within transcribed loci ( Supplementary Table 4 ). Given the limited species distribution and high-sequence identity between genomic GAS5 sequences and these copies, the retrotransposition events described here are relatively recent. It is likely that additional, ancient copies of GAS5 are present in mammalian genomes but have diverged beyond recognition. Using a range of structural and biochemical approaches, we offer a mechanism to explain the potent ability of Gas5 to suppress SR-mediated transactivation. This repression is mediated through sequence-specific protein RNA-contacts within an A-form double helical structure with a widened major groove that facilitates SR binding. We show that full-length, fully spliced Gas5 binds strongly to the GR DBD, with affinity comparable to physiological DNA GREs [23] . In addition, GR exhibits stronger binding to full-length Gas5 than single (+)GRE half-sites or the newly characterized negative GREs [26] , [39] , illustrating the strength of the GR–Gas5 interaction as well as the versatility of GR as a diverse nucleic acid-binding protein [23] , [40] , [41] . GR is one of a growing number of proteins that bind DNA and RNA, a class that includes ADAR, TFIIIA and the p50 subunit of nuclear factor-κB, among many others [42] . p50 has been crystallized in complex with its DNA response element as well as a competing RNA aptamer [43] , [44] . The RNA aptamer adopts a similar conformation as nuclear factor-κB response elements, and p50 makes nearly identical contacts with RNA as it does with DNA [43] ; we expect a similar mechanism of DNA mimicry occurs with GR and Gas5. Here we show that GR–Gas5 interactions are mediated through helix 1 of GR’s DBD, demonstrating that GR uses the same surface to bind both DNA and Gas5 RNA. However, the dimerization loop of the GR DBD is not affected upon Gas5 binding, although more study is required to definitively determine GR’s dimerization status when bound to RNA, given recent reports demonstrating the importance of the ligand-binding domain in receptor dimerization [45] . Although the exact Gas5 GREM sequence does not appear in any human mRNAs, we have demonstrated that this sequence evolved from a splice acceptor site; therefore, GR may be able to recognize RNA transcripts similar to Gas5 at splice site sequences; GR has been previously shown to affect the alternate splicing of several genes [46] , [47] , [48] . The potent repression of SR signalling by Gas5 is likely explained by both the strong affinity of the SR-Gas5 interaction and by the large discrepancy between Gas5 copy number and GR DNA-binding sites in a cell during periods of Gas5 upregulation. In HeLa cells, Gas5 copy number increases by an order of magnitude to roughly 75,000 during serum starvation [14] , which is on par with or greater than the increase in Gas5 expression caused by exogenous transfection in this study ( Fig. 5a,d,g ). In contrast, available genomic GR-binding sites are roughly fixed in number, ranging from 3,000 to 8,000 depending on cell type [35] . This suggests that Gas5 regulates SR activity by simply titrating its own GR-binding site against genomic GR-binding sites. However, it is unclear whether Gas5 interferes with DNA binding-independent, SR-mediated transrepression such as ‘tethered’ GR transrepression [49] . Future studies are needed to determine if Gas5 modulates these DNA-independent effects. The GAS5 gene is unique in its high level of alternative splicing: at least 29 non-redundant, alternatively-spliced transcripts originate from the GAS5 locus [15] , making it one of the most highly alternatively spliced genes in the genome. Although it is not clear whether Gas5 splicing patterns are tissue-specific, the majority of Gas5 splice variants include the GREM, which is sufficient for SR binding. Notably, we recently showed that exon 12-containing Gas5 transcripts are downregulated in breast ductal carcinoma compared with adjacent normal tissue [21] . Nevertheless, 13 Gas5 splice variants either exclude exon 12 or shorten exon 12 such that the GREM is not included in the final transcript [50] , indicating that alternative splicing may present an additional level of SR regulation by Gas5. Such control may be required for tissue-specific homeostasis and may be disrupted by single-nucleotide polymorphisms (SNPs) that affect the splicing of GREM-containing exon 12 (rs11537772, rs111755386). An additional SNP that alters the GREM sequence (G559U) has also been described (rs186249529). Mutation of G559 in this study, even when combined with a compensatory mutation to preserve secondary structure, dramatically weakens the GR–Gas5 interaction ( Fig. 4e ), potentially attenuating riborepression of SR signalling. Thus, it is possible these and other Gas5 SNPs may predispose individuals to steroid-driven cancers despite apparently normal tissue levels of Gas5. Given the paucity of identified sequence-specific lincRNA function, we used the detailed biochemical and structural data here to examine the evolutionary origin of the Gas5 GREM. The SR DBDs are highly conserved throughout vertebrates; in contrast, two recent studies with lincRNA functional domains show mixed levels of conservation: megamind and cyrano show conserved function between zebrafish and mammals [12] , whereas key functional human domains of the lincRNA HOTAIR are missing in mice [51] . Given the comparatively faster sequence turnover within lincRNAs compared with their protein targets, we propose that Gas5 co-opted a splice acceptor site into its current SR-binding role. Such a mechanism allows the primary sequence required for SR binding to be conserved because of the presence of a second, stronger pressure for conservation. The relatively loose sequence requirements of an acceptor splice site—a polypyrimidine tract followed by AG—may have allowed this locus to gradually acquire SR-binding ability in eutherian mammals ( Supplementary Fig. 5d ). However, it is clear that once Gas5-SR binding was established, this function was conserved, given the retention of splice site-like sequences required for SR binding at the GREM ( Fig. 7c ). The development of this functional domain within the translationally regulated 5′ terminal oligo-pyrimidine Gas5 transcript may have provided an important link between translational downregulation and other critical events involved in growth arrest [18] . Given the large number—tens of thousands—of lincRNAs, it is likely that hundreds of lincRNAs have precise, sequence-specific functions analogous to that of Gas5. Furthermore, given their large size, it is likely that some lincRNAs contain multiple protein-recognition sites and may serve as scaffolds for protein complexes. Here we have demonstrated that the interaction between Gas5 and SRs depends on unique structural elements and precise, sequence-specific interactions to differentiate among target proteins. Subtle disruptions of these interactions have dramatic effects on cell fate. Further, we show that the lincRNA Gas5 co-opted splicing regulatory sequences into a SR-binding role, explaining functional and sequence conservation at the GREM. Together, these results demonstrate that lincRNAs can contain conserved, sequence-specific protein interaction surfaces that ensure a high level of specificity to bind to target proteins and control cell fate. Protein expression and purification The DBDs of the human GR (GenBank ADP91253.1; residues L381-E541), AR (UniProtKB P10275.2; residues D550-K630), PR (UniProtKB P06401.4; residues E560-F642), MR (GenBank AAA59571.1; residues S593-G671) and ER (UniProtKB P03372.2; residues A175-R260) were cloned as 6X Histidine fusions into the pMCSG7 vector. Mutations were made with the QuikChange site-directed mutagenesis kit (Stratagene). The DBDs were expressed based on previous protocols [26] , [52] : transformed BL-21(DE3)pLysS Escherichia coli were induced with 0.3 mM isopropyl-β- D -thiogalactoside for 4 h at 30 °C. Cells were lysed in 1 M NaCl, 20 mM Tris-HCl, pH 7.4, 25 mM imidazole, 5% glycerol via sonication, and protein was purified via affinity chromatography (HisTrap) followed by TEV protease cleavage and dialysis to 100 mM NaCl, 20 mM Tris-HCl, pH 7.4, 25 mM imidazole and 5% glycerol. The DBDs and tags were separated by affinity chromatography (HisTrap), and further purified by gel filtration chromatography. For storage, protein was concentrated to 4 mg ml −1 , flash frozen in liquid N 2 and stored at −80 °C. For 15 N labelling, the GR DBD was expressed in M9 minimal media with 15 NH 4 Cl as the nitrogen source. Cultures were inoculated at an OD 600 of 0.3–0.4, and induced for 14 h with 1 mM isopropyl-β- D -thiogalactoside at an OD 600 of 1.2. The GR DBD was then purified via affinity chromatography as above. Nucleic acid synthesis and purification Constructs for in vitro transcription were ligated into the puc57 vector using a forward primer with the T7 promoter sequence and a reverse primer using the Hin dIII restriction site. Plasmid was cut overnight with Hin dIII (Fermentas) and used as template for in vitro transcription in 50 mM Tris-HCl, pH 7.5, 15 mM MgCl 2 , 5 mM DTT and 2 mM spermidine with 2 mM each of individual nucleoside triphosphates. Recombinant T7 RNA polymerase (0.1 mg ml −1 per reaction) and inorganic pyrophosphatase (1 U ml −1 per reaction, Fermentas) were added and the reaction was incubated for 5 h at 37 °C. RNA was purified by anion exchange chromatography as described previously [53] and ethanol precipitated. Both in vitro transcribed and synthetic nucleic acid duplexes (Integrated DNA Technologies) were annealed in 10 mM NaCl, 20 mM Tris-HCl, pH 8.0, by heating to 85 °C and slow cooling to room temperature. Nucleic acid-binding assays FP was used to detect the formation of DBD-nucleic acid complexes. Indicated amounts of DBD were added to wells containing 10 nM of 5′ carboxyfluorescein-labeled nucleic acids. For competition assays, labelled DNA was used at a concentration 1.2 times higher than the GR–(+)GRE K d . Reactions were performed in 100 mM NaCl, 20 mM Tris-HCl, pH 7.4, 5% glycerol and measured with a Biotek Synergy plate-reader (BioTek) at an excitation/emission wavelength of 485/528 nm. FP data were analysed and graphed using GraphPad Prism 5 (Graphpad Software, Inc.). Error is shown as ±s.e.m., and was normalized to the mean for figures showing –logK d . Sequences used in binding experiments can be found in Supplementary Fig. 1 . All binding experiments were performed at least in duplicate, with three internal replicates. Ultraviolet melting assays Ultraviolet melting assays were conducted as described previously [54] . Briefly, samples containing 25 μg RNA in a solution of 10 mM Tris, pH 7.4, and 20 mM NaCl were melted and ultraviolet absorption collected on a Varian Cary 400 ultraviolet–visible spectrophotometer. Sample temperatures were measured with an in-cell temperature probe. First derivatives of the melting curves were calculated in GraphPad Prism 5. Hydroxyl radical probing In vitro transcribed Gas5 GREM RNA was treated with FastAP (Fermentas) and 5′-end labelled using [γ- 32 P]ATP and T4 polynucleotide kinase. Labelled RNA was urea denaturing gel purified and annealed by heating at 65 °C for 10 min and slowly cooling to room temperature before use. GR was dialysed against 20 mM Tris, pH 7.5, 100 mM NaCl. In a total volume of 25 μl, labelled RNA (50,000 c.p.m.) was incubated without or with GR (0.2, 0.8, 3 or 12 μM) and hydroxyl radicals produced by adding 1 μl each of 50 mM Fe(SO 4 ) 2 , 100 mM EDTA, 250 mM ascorbic acid and 3% (v/v) hydrogen peroxide. The reaction was allowed to proceed on ice for 5 min before quenching by ethanol precipitation in the presence of yeast tRNA (0.4 mg ml −1 ) as a carrier and resolving the RNA products by 12% urea denaturing-polyacrylamide gel electrophoresis for 1.5 h at 55 W. Control experiments with labelled RNA and GR were preformed to ensure no contaminating RNases were present in the E. coli -expressed protein. Band quantification was performed with ImageQuant applying the Rubber Band background subtraction. For normalization, the intensity of each band was measured and normalized to the most intense band in 0 μM GR. The normalized intensities were compared between 0 and 12 μM GR. A nucleotide was considered strongly protected/enhanced if the difference in normalized intensity was greater (±) 20%, or moderately protected if the difference was 10%. Crystallization and structure analysis Bipyramidal crystals of the Gas5 GREM duplex appeared in two conditions. Crystals grown in 0.05 M sodium succinate, pH 5.5, 0.5 mM spermine, 0.02 M MgCl 2 and 3 M ammonium sulfate were frozen directly in liquid N 2 . Data from these crystals were collected at 100 K at the Emory University home source to a resolution of 2.2 Å at a wavelength of 1.54 Å. Crystals that formed in 0.1 M citric acid, pH 4, and 3 M ammonium sulfate were cryoprotected in 0.1 M citric acid, pH 4, 3 M ammonium sulfate and 10% glycerol and flash-frozen in liquid N 2 . Data from these crystals were collected at the Advanced Photon Source BM-22 at a wavelength of 1.00 Å, and data from both crystals were integrated and indexed in HKL-2000. Phases were determined using molecular replacement from an ideal RNA helix modelled in Coot [55] , using PHASER in the PHENIX suite [56] . Crystal twinning was detected using phenix.xtriage, and twin refinement was performed in phenix.refine [56] . Molprobity indicated no incorrect sugar puckers, bad bonds or bad angles in both crystal structures. The composite omit map utility within PHENIX was used to generate the simulated annealing composite omit map [56] . Representative electron density is shown in Supplementary Fig. 7 . RNA and DNA structure analyses were performed in 3DNA [57] , using refined P-P distances to determine major and minor groove widths. Figures of models and crystal structures were generated in the PyMOL Molecular Graphics System (Schrödinger LLC). NMR NMR data were collected at 25 °C on a Bruker 700 MHz 1 H frequency equipped with a QCI cryoprobe. For RNA NMR experiments, the 33 nt Gas5 RNA ( Supplementary Fig. 1 ) was reconstituted after ethanol precipitation in 20 mM phosphate, 50 mM KCl, 10% D 2 O buffer, pH 7.4 to a final concentration of 10 mg ml −1 . The RNA sample was annealed by denaturing at 95 °C for 5 min and equilibrating to room temperature (20–23 °C) overnight. Two-dimensional 1 H-detected NOESY and total correlation spectroscopy spectra were collected using 100- and 200-ms mixing times for Gas5 RNA and after adding equimolar concentration of GR DBD. The proton carrier frequency was set coincident with the water resonance for all experiments. For protein NMR experiments, 2D [ 1 H, 15 N]-HSQC spectra were collected for free 15 N-labelled GR DBD protein or complexed with 33 nt Gas5 RNA in the same buffer as above. Chemical shift perturbations were assigned using previously published GR DBD NMR chemical shifts [29] and calculated using the minimum chemical shift perturbation procedure [58] . Data were analysed with NMRViewJ (OneMoon Scientific, Inc.) [59] . Modelling of the GR DBD-Gas5 RNA complex NMR chemical shift perturbation and mutagenesis data were used as input to HADDOCK [31] to model the GR DBD-Gas5 RNA complex. Before docking, the AMBER 12 package [60] was used to perform molecular dynamics on the crystal structure of the Gas5 GREM duplex in order to widen the major groove. Briefly, the tleap module was used to solvate the Gas5 GREM using a TIP3P octahedral box water model [61] and neutralize the system. The ff12SB force field was employed in the calculations with the sander module used for the equilibration period and the pmemd.cuda code [62] , [63] used on a graphics processor unit for the production runs. The system was equilibrated in a multi-step process [64] , starting with 10,000 steps of energy minimization (5,000 steps of steepest descent, followed by 5,000 steps of conjugate gradient); all non-water and non-hydrogen atoms were restrained during this minimization step. The systems were then equilibrated for 200 ps in the canonical NVT ensemble [65] during which time the temperature was ramped from 10–295 K during the first 100 ps and the restraints on the solute atoms were retained. Particle-MESH-Ewald periodic boundary conditions and a cutoff of 1 nm for both electrostatic and Lennard-Jones interactions were employed; the SHAKE algorithm [66] was applied to constrain bonds to hydrogen atoms, and a time step of 1 fs was used. After HADDOCK docking, the lowest energy docked model from the best scoring cluster was used as the representative model. Statistics for the highest scoring cluster are presented in Supplementary Table 5 . Cell culture Human adherent cell lines, 22Rv1 (prostate carcinoma cells) and MCF-7 (breast carcinoma cells), and suspension cell lines, Jurkat, CEM-C7 (both T-lymphoblastic leukemia cells) and JeKo-1 (Mantle cell B lymphomacells) were routinely cultured in R-10 medium (RPMI-1640 medium supplemented with L -glutamine (2 mM), fetal bovine serum (10%) and gentamicin (50 μg ml −1 )) at 37 °C in a humidified incubator with 5% CO 2 . CEM-C7 and Jurkat cells were derived from ref. 67 , the 22Rv1 cells used are an apoptosis-sensitive clone described in ref. 68 , MCF-7 cells were purchased from American Type Culture Collection and JeKo1 cells were a gift of Dr. Aneela Majid. For experiments to determine the influence of Gas5 on androgen signalling, 22Rv1 cells were switched to prf R-10 DCSS (phenol red-free RPMI-1640 medium supplemented with L -glutamine (2 mM), dextran charcoal-stripped fetal bovine serum (10%) and gentamicin (50 μg ml −1 )) at 24 h before transfection. All experiments were carried out using cells in the logarithmic phase of growth. Plasmid DNA transfection WT Gas5 (NR_002578.2 bases 1–631) was cloned into the pcDNA3.1 vector and the G549A mutation made with the Quikchange site-directed mutagenesis kit (Stratagene). 22Rv1, MCF7 cells (each at 2 × 10 6 cells in 0.1 ml Nucleofector solution V) and JeKo-1 cells (5 × 10 6 cells in 0.1 ml Nucleofector solution R) were nucleofected with 2 μg plasmid, using programmes X-001, E-014 and X-001, respectively. Cells were diluted to 2 ml with R-10 medium (or prf R-10 DCSS medium, as appropriate) and cultured in six-well plates. Determination of apoptosis and cell survival Adherent cell lines were trypsinized at 24 h post -nucleofection, samples were collected for RNA isolation, and cells were re-plated in 12-well plates (8 × 10 4 cells per well). For 22Rv1 and MCF-7 cells, additional samples were irradiated with ultraviolet light to induce apoptosis before re-plating: cells (10 5 per ml medium) in plastic Petri dishes (lids removed) were exposed to a dose of 40 J m −2 ultraviolet-C light, then immediately centrifuged and resuspended in fresh medium. After culture for 24 h (22Rv1) or 48 h (MCF7), cells were trypsinized, and adherent and non-adherent cells were combined. Suspension cell lines were also collected at 24 h following transfection for total RNA isolation and for re-plating at 2 × 10 5 cells per well in 12-well plates. To determine viability, cells were stained with 0.1% nigrosin (w/v) and counted using a haemocytometer; cells which excluded the dye were considered to be viable. To determine apoptosis, cells were stained with acridine orange (25 μg ml −1 ), and the proportion of cells containing condensed or fragmented chromatin was scored by fluorescence microscopy (≥200 cells per treatment were scored). In some experiments, the proportion of cells containing activated caspase activity was determined using a commercial Caspatag assay (CaspaTag Pan-Caspase In Situ Assay Kit, Millipore) and fluorescence microscopy (≥200 cells per treatment were scored), according to the supplied instructions. Clonogenic assay Long-term survival and proliferation of transfected JeKo-1, CEM-C7 and Jurkat cells were assessed by the ability of the cells to form colonies in soft agar. An equal proportion of the culture from each experimental condition was diluted in 5 ml Iscove’s medium (Sigma) containing 20% heat-inactivated fetal calf serum, 10% cell conditioned medium and 0.3% Noble agar (Difco) and plated in 60 mm dishes. Dishes were also overlaid with 2.5 ml Iscove’s complete medium containing 10% cell conditioned medium. The number of colonies formed was counted following 2–3 weeks incubation at 37 °C in 5% CO 2 . Determination of androgen sensitivity 22Rv1 cells were trypsinized at 24 h post -nucleofection and cells were re-plated in 12-well plates (8 × 10 4 cells per well) in prf R-10 DCSS . Cells were allowed to attach to plates for 6 h, then treated with 10 nM R1881 in prf R-10 DCSS ; controls received 0.05% DMSO. After 4 h, cells were collected in TRIZOL reagent (Invitrogen) for total RNA isolation. Real-time PCR analysis of gene expression Total RNA was isolated using TRIZOL reagent (Invitrogen), treated with RQ1 RNase-free DNase (Promega) then reverse transcribed using random hexamer priming and SuperScript II Reverse Transcriptase (Invitrogen), according to the supplied protocols. For determination of Gas5 levels, real-time PCR was conducted using SensiFast Probe Hi-ROX kit (Bioline) and Taq Man Gene Expression Assays (Applied Biosystems; assay codes Hs03464472_m1 for GAS5 and Hs99999901_m1 for 18S). For determination of expression levels of androgen-responsive genes, real-time PCR was conducted using SensiFast SYBR Hi-ROX kit (Bioline) according to the supplied instructions and primer sets specific for: KLK2 (forward: 5′-ATGTGTGCTAGAGCTTACTC-3′; reverse: 5′-AAGTGGACCCCCAGAATCAC-3′); KLK3 (forward: 5′-CCAAGTTCATGCTGTGTGCT-3′; reverse: 5′-CCCATGACGTGATACCTTGA-3′); FKBP5 (forward: 5′-CGCAGGATATACGCCAACAT-3′; reverse: 5′-GAAGTCTTCTTGCCCATTGC-3′) and ACTB (forward: 5′-GTTTGAGACCTTCAACACCC-3′; reverse: 5′-ATGTCACGCACGATTTCCC-3′). Assays contained 10 ng sample cDNA in a final volume of 25 μl and were run on an ABI Prism Sequence Detection System model 7000. For adherent cell lines, standard curves, comprising 0.2–60 ng cDNA (prepared from parental cells), were included with each assay to allow relative quantifiation; standard curves of threshold cycle ( C T ) value versus log input standard cDNA were constructed by linear regression, and the equation of the line was used to calculate input amounts of samples from their respective C T values. For suspension cell lines, quantitation of Gas5 was determined using the comparative C T method, using parental cells as calibrators. Gas5 levels were expressed relative to 18S rRNA, and levels of androgen-responsive genes were expressed relative to ACTB. Evolutionary analysis Genomic sequences of the GAS5 locus were downloaded from the Ensembl database [50] . For species where Gas5 was not annotated, the exon 12 sequence was determined using splice prediction downstream of SNORD81 (ref. 69 ). Sequences were aligned in Geneious (Biomatters), and evolutionary rate analysis was conducted with the haplorhine sequences in MEGA 5 with the Tamura-Nei model, using all sites and three gamma rate categories [70] . Accession codes: The Gas5 GREM duplex crystal structures have been deposited to the PDB under accession numbers 4MCE and 4MCF . How to cite this article : Hudson, W. H. et al. Conserved sequence-specific lincRNA-steroid receptor interactions drive transcriptional repression and direct cell fate. Nat. Commun. 5:5395 doi: 10.1038/ncomms6395 (2014).